Metal ion-directed dynamic splicing of DNA through global conformational change by intramolecular complexation Chemically engineered DNAs—in which global conformation can be modulated in response to specific stimuli—could be allosteric functional DNAs themselves or work as a modulator of the functional nucleic acids such as DNAzymes and aptamers. Here, we show that two terpyridines built in the DNA backbone form a stable intramolecular 1:2 complex, [M(terpy) 2 ] 2+ , with divalent transition metal ions. Upon complexation, the DNA conjugates adopt a Ω-shape structure, in which two distal sequences located outside the terpyridines connect with each other to form a continuous segment with a specific structure or sequence. Such a DNA structure is globally controlled by local metal complexation events that can be rationally designed based on general coordination chemistry. This method is regarded as metal ion-directed dynamic sequence edition or DNA splicing. DNAzymes with peroxidase-like activity can thus be regulated by several transition metal ions through sequence edition techniques based on the Ω-motif. Recently, several research groups have reported on the fabrication of specific DNA structures using metal ion-directed techniques [1] , [2] , [3] , [4] , [5] , [6] , [7] , [8] , [9] , [10] , [11] , [12] , [13] , [15] , [16] , [17] , [18] , [19] , [20] , [21] . For example, two thymines and cytosines coordinate to Hg 2+ and Ag + , respectively, to form a M-DNA (metal ion DNA complex) duplex through the formation of metal-centred nucleobase dimers [7] , [8] , [12] , [13] , [15] . A silver ion can be accommodated in the nucleobase triplet CGC of a DNA triplex by substitution of the N3 proton of cytosine on the third strand, which stabilizes the triplex structure even under neutral pH [10] , [11] . The knowledge of the specific coordination of nucleobases to these soft metal ions enabled us to prepare stable duplexes or triplexes by designing the sequences. On the other hand, several DNA analogues carrying metal chelators instead of natural nucleobases have been reported. Chelators, such as catechol, phenylenediamine, aminophenol and hydroxypyridone, selectively coordinate to certain transition metal ions to form stable M-DNA duplexes or triplexes [4] , [5] , [6] . The DNA conjugates with chelator molecules on their backbone have also been reported to form unique structures [9] , [16] , [17] , [18] , [19] , [20] , [21] . In the past decade, a number of functional nucleic acids, such as ribozymes, DNAzymes and aptamers, have been isolated using techniques of molecular evolution [22] , [23] . These nucleic acids have been applied to analytical systems for various biomolecules as functional modules for analyte recognition and signal amplification [24] , [25] , [26] , [27] . Prescribed higher-ordered structures are critically important for these nucleic acids to express their intrinsic functions. Therefore, techniques that control formation of their structures should be useful to modulate their functions. If the chemical groups, which respond to certain stimuli by changing their structure, are incorporated into the backbone of the functional DNAs or their complementary sequences, we could regulate their functions by controlling conformational changes in the DNAs. This strategy is general in the sense that it targets the higher-ordered structure of functional nucleic acids rather than each of their particular functions themselves. The techniques for drastic changes in DNA conformation could also be applied to regulate gene expression by certain stimuli such as decoy, antisense and RNAi strategies. Herein, we synthesized 2,2′:6′,2′′-terpyridine (terpy)-based amidite reagents. Terpy units can be incorporated into any positions in the DNA backbone with these amidite reagents using automated DNA synthesis. Terpy forms a stable complex with Fe 2+ and some other divalent transition metal ions [28] , [29] . We expected that the stiffness and conformation of the DNA backbone could be controlled through complexation with certain metal ions. Then, it would enable us to regulate the activity of functional nucleic acids. We have already reported the effect of metal ions on the stability of DNA structures consisting of the conjugates with one terpy (synthesized using 1 mentioned below). The terpy incorporated in the stem moiety of the duplex stabilized the structure by complexation, which confers entropic benefit on the DNA. In contrast, the structure of bimolecular triplexes carrying a terpy unit in its loop moiety significantly destabilizes on complexation with divalent transition metal ions [30] . This can be explained by the change in the length of the terpy unit in the loop of the triplex by metal coordination; the metal-bound terpy connecting two pyrimidine strands is too short to cap the base triplet in the structure of the DNA triplex. In the present study, two terpy units are incorporated into the backbone of a DNA strand to form terpy 2 –DNA conjugates, in which two terpys are located at distant positions from each other with an intervening sequence. It is expected that transition metal ions, such as Fe 2+ , forms a 1:2 complex with the two terpys in a terpy 2 –DNA conjugate. To form such an intramolecular complex, the backbone of terpy 2 –DNA conjugates make adopt an Ω-shaped conformation, where the two distal sequences outside both terpys in the sequence are directly connected with each other to form a continuous stretch of the specific structure or sequence. Such global conformational control of DNA would be regarded as metal ion-directed sequence edition or reversible splicing of DNA. We perform allosteric regulation of catalytic activity of DNAzyme through metal ion-directed sequence edition of DNA. DNA preparation and system design In this study, we aimed to regulate the function of DNAzyme with peroxidase-like activity [31] , [32] by conformational control of the terpy 2 –DNA conjugate. To incorporate terpy units into the backbone of the DNA, terpy-based amidite reagents were prepared. We synthesized two amidite reagents 1 and 2 ( Fig. 1a ) according to the schemes shown in Supplementary Information . Although both of them have a 2,2′:6′,2′′-terpyridine structure with two ethylene linker chains connecting to phosphoramidite and dimethoxytrityl-protected hydroxyl groups, the substitution position of the linkers are different. 1 and 2 tether the two linker chains from 6,6′′- and 5,5′′-positions of terpy, respectively. 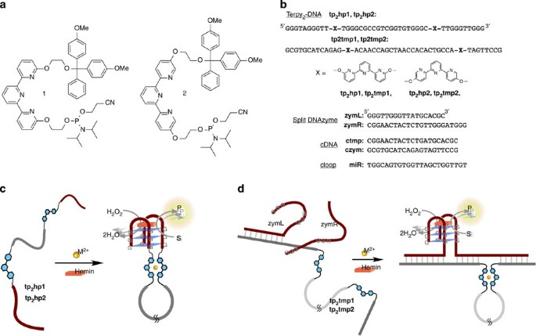Figure 1: DNA structures, sequences and constructions of allosteric DNAzymes. (a) Structures of terpyridine-based amidite reagents,1and2. (b) Sequences of terpy2–DNA conjugates and DNAs used in this study. (c) Working principle of metal ion-dependent DNAzyme,tp2hp1andtp2hp2. The modified DNAzyme adopts an active hairpin structure by intramolecular metal complexation. (d) Allosteric regulation of split DNAzyme activity by metal ion-directed dynamic sequence edition of the template,tp2tmp1andtp2tmp2. Figure 1: DNA structures, sequences and constructions of allosteric DNAzymes. ( a ) Structures of terpyridine-based amidite reagents, 1 and 2 . ( b ) Sequences of terpy 2 –DNA conjugates and DNAs used in this study. ( c ) Working principle of metal ion-dependent DNAzyme, tp 2 hp1 and tp 2 hp2 . The modified DNAzyme adopts an active hairpin structure by intramolecular metal complexation. ( d ) Allosteric regulation of split DNAzyme activity by metal ion-directed dynamic sequence edition of the template, tp 2 tmp1 and tp 2 tmp2 . Full size image The sequences of the DNAs used in this study are shown in Fig. 1b . The four terpy 2 –DNA conjugates, tp 2 hp1 , tp 2 hp2 , tp 2 tmp1 and tp 2 tmp2 , were prepared using 1 and 2 according to the standard phosphoramidite method shown in Supplementary Information . The last letter in the names of the terpy 2 –DNA conjugates, ‘1’ or ‘2’, stands for the amidite reagents 1 and 2 built in their sequences, respectively. We designed two systems for regulation of oxidation reactions by DNAzyme. In one system, we used the modified DNAzyme, tp 2 hp1 and tp 2 hp2 , which can adopt a hairpin form by intramolecular metal complexation. The sequence of DNAzyme was split into two parts [33] , and each half was attached to both ends of a part of the complimentary sequence of the H- ras gene [34] through terpys to form tp 2 hp1 and tp 2 hp2 . The catalytic activity of tp 2 hp1 and tp 2 hp2 were expected to be restored when forming a hairpin conformation induced by intramolecular 1:2 metal complexation ( Fig. 1c ). Reconstruction of an integrated active DNAzyme on the allosteric template, tp 2 tmp1 and tp 2 tmp2 , was expected in another system. The same DNAzyme mentioned above was also split into two parts, and then the short binding arms were attached to the end of these parts to form a pair of the half DNAzymes [33] , zymR and zymL . The outside two sequences in tp 2 tmp1 and tp 2 tmp2 were designed to be complementary to the binding arms of zymR and zymL . Therefore, tp 2 tmp1 and tp 2 tmp2 are expected to work as an effective template when both outside sequences come in proximity with each other by forming an Ω-shaped conformation through 1:2-type intramolecular metal complexation ( Fig. 1d ). The loop sequences between the two terpys of tp 2 tmp1 and tp 2 tmp2 are designed to be complementary to miR-34 (microRNA) [35] . Preliminary studies of complexation Complexation of the terpy 2 –DNA conjugates, tp 2 tmp1 and tp 2 tmp2 , with metal ions were investigated by ultraviolet–visible (vis) titrations. Four divalent transition metal ions, Fe 2+ , Ni 2+ , Cu 2+ and Zn 2+ , were used in this study ( Fig. 2 ). The aliquots of transition metal ions were added into the conjugate solutions, and their ultraviolet–vis spectrum was recorded after each addition. The spectral changes and the plots of absorbance around the peak with Fe 2+ titration are shown in Fig. 2a,b . The complexation behaviour of the two conjugates was completely different. tp 2 tmp1 showed stoichiometric complexation with Fe 2+ . The absorbance increased monotonously and saturated at the point of [Fe 2+ ]/[ tp 2 tmp1 ]=2.0 ( Fig. 2a ), indicating that each of the two terpys on a tp 2 tmp1 bound a Fe 2+ to form two [Fe(terpy)] 2+ on a tp 2 tmp1 . In contrast, the stoichiometry of tp 2 tmp2 complexation was clearly shown to be 1.0 (=[Fe 2+ ]/[ tp 2 tmp2 ]) ( Fig. 2b ), indicating that the terpy units formed [Fe(terpy) 2 ] 2+ on tp 2 tmp2 . Further change was not observed in the spectra even with more additional Fe 2+ . The characteristic band was observed at 530 nm. This is attributed to the metal-to-ligand charge-transfer band of the 1:2 complex, [Fe(terpy) 2 ] 2+ (refs 28 , 29 ). Interestingly, this meant that the complex [Fe(terpy) 2 ] 2+ did not form on tp 2 tmp1 but exclusively formed on tp 2 tmp2 . All of the results observed in the ultraviolet–vis titrations were reproduced in the presence of the complementary DNA, ctmp , which is the tandem sequence complementary to the two distal sequences outside of the two terpys. 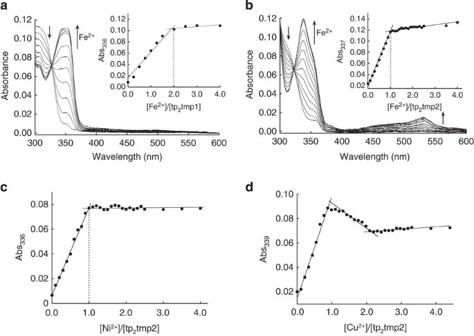Figure 2: Preliminary spectrophotometric studies for metal complexation of tp2tmp1 and tp2tmp2 with divalent transition metal ions. (a) Spectral change oftp2hp1in ultraviolet–vis titration of Fe2+. Inset: the absorbance at 356 nm was plotted against the feeding ratio, [Fe2+]/[tp2hp1]. (b) Spectral change oftp2hp2in ultraviolet–vis titration of Fe2+. Inset: the absorbance at 337 nm was plotted against the feeding ratio, [Fe2+]/[tp2hp2]. (c) The result of Ni2+titration. The absorbance at 336 nm was plotted against the feeding ratio, [Ni2+]/[tp2hp2]. (d) The result of Cu2+titration. The absorbance at 339 nm was plotted against the feeding ratio, [Cu2+]/[tp2hp2]. The titrations were performed with 2.0 μM DNA in HEPES buffer solution (10 mM, pH 7.0) containing 500 mM NaCl at 25 °C. Figure 2: Preliminary spectrophotometric studies for metal complexation of tp 2 tmp1 and tp 2 tmp2 with divalent transition metal ions. ( a ) Spectral change of tp 2 hp1 in ultraviolet–vis titration of Fe 2+ . Inset: the absorbance at 356 nm was plotted against the feeding ratio, [Fe 2+ ]/[ tp 2 hp1 ]. ( b ) Spectral change of tp 2 hp2 in ultraviolet–vis titration of Fe 2+ . Inset: the absorbance at 337 nm was plotted against the feeding ratio, [Fe 2+ ]/[ tp 2 hp2 ]. ( c ) The result of Ni 2+ titration. The absorbance at 336 nm was plotted against the feeding ratio, [Ni 2+ ]/[ tp 2 hp2 ]. ( d ) The result of Cu 2+ titration. The absorbance at 339 nm was plotted against the feeding ratio, [Cu 2+ ]/[ tp 2 hp2 ]. The titrations were performed with 2.0 μM DNA in HEPES buffer solution (10 mM, pH 7.0) containing 500 mM NaCl at 25 °C. Full size image The only difference between tp 2 tmp1 and tp 2 tmp2 is the tethering positions of the terpys connected to DNA backbones. We calculated the structures of both complexes using the density functional theory (DFT) method (B3LYP/6-31G*). The optimized structures of [Fe(terpy) 2 ] 2+ are shown in Fig. 3 . The structure of Fig. 3a is the complex consisting of a Fe 2+ and two 6,6′′-tethered terpys and Fig. 3b is of a Fe 2+ and two 5,5′′-tethered terpys, each of which is the complex expected to form on tp 2 tmp1 (or tp 2 tmp1/ctmp ) and tp 2 tmp2 (or tp 2 tmp2/ctmp ), respectively. In the structure of [Fe(terpy) 2 ] 2+ with 6,6′′-tethered terpys, the linker chains on a terpy almost touches the central pyridine ring of another terpy in the complex. This steric hindrance should make the complex unstable or impossible to form. In contrast, this hindrance was not observed in the complex consisting of 5,5′′-tethered terpys. This would explain the difference in complexation behaviour between tp 2 tmp1 and tp 2 tmp2 observed in ultraviolet–vis titration. 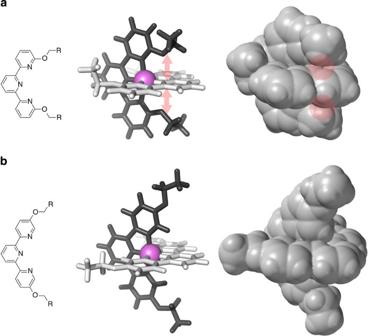Figure 3: Optimized structures of [Fe(terpy)2]2+with 6,6′′-substituted and 5,5′′-substituted terpyridines. Both structures were optimized with DFT calculation (B3LYP/6-31G*). (a) Optimized structure of [Fe(terpy)2]2+with 6,6′′-terpyridines, which is proposed to form ontp2hp1andtp2tmp1. (b) Optimized structure of [Fe(terpy)2]2+with 5,5′′-terpyridines, which is proposed to form ontp2hp2andtp2tmp2. The two structures shown in the centre and the right-hand side are different representations of the same structures, stick model and Van der Waals surface, respectively. Figure 3: Optimized structures of [Fe(terpy) 2 ] 2+ with 6,6′′-substituted and 5,5′′-substituted terpyridines. Both structures were optimized with DFT calculation (B3LYP/6-31G*). ( a ) Optimized structure of [Fe(terpy) 2 ] 2+ with 6,6′′-terpyridines, which is proposed to form on tp 2 hp1 and tp 2 tmp1 . ( b ) Optimized structure of [Fe(terpy) 2 ] 2+ with 5,5′′-terpyridines, which is proposed to form on tp 2 hp2 and tp 2 tmp2 . The two structures shown in the centre and the right-hand side are different representations of the same structures, stick model and Van der Waals surface, respectively. Full size image The stoichiometry of Ni 2+ – tp 2 tmp2 complexation was almost the same with Fe 2+ mentioned above ( Fig. 2c , spectral change: see Supplementary Fig. 1 ). That is, regardless of the feeding ratio, [M 2+ ]/[ tp 2 tmp2 ], Fe 2+ and Ni 2+ seem to form a rather stable complex, [M(terpy) 2 ] 2+ , on tp 2 tmp2 . Meanwhile, Cu 2+ ( Fig. 2d , spectral change: see Supplementary Fig. 2 ) and Zn 2+ (see Supplementary Fig. 3 ) showed a multiphasic unique spectral change. For both titrations, two apparent inflection points were observed at [M 2+ ]/[ tp 2 tmp2 ] ratios of 1.0 and 2.0, indicating that the two types of complexes with different stoichiometry were successively formed with the addition of the metal ions. 1:2 complex, [M(terpy) 2 ] 2+ , formed on tp 2 tmp2 at a lower feeding ratio, which changed to a 1:1 complex, [M(terpy)] 2+ upon further addition of metal ions. The difference in the stoichiometry of the complexes of the four transition metal ions could be explained by the relative magnitude of successive binding constants, K 1 and K 2 ; Fe 2+ : log K 1 =7.1, log K 2 =13.8; Ni 2+ : 10.7, 11.2; Zn 2+ : 6.7, 5.2; Cu 2+ : 13.0, not available (that is, K 2 is much smaller than K 1 ). Whereas the magnitudes of K 1 are larger than K 2 for Fe 2+ and Ni 2+ , the opposite is true for Cu 2+ and Zn 2+ (refs 28 , 36 ). To identify the complex, an equimolar mixture of terpy 2 –DNA and Fe 2+ was subjected to matrix-assisted laser desorption ionization time-of-flight mass spectrometry. The short terpy 2 –DNA conjugate (18-mer DNA conjugate carrying two terpy units) was prepared for this study using the terpy amidite 2 . Using the conjugate with a lower molecular weight, we can obtain accurate and precise m / z values of the complexes, even for multimeric DNAs. The result are shown in Supplementary Fig. 4 . The only complex observed was [terpy 2 –DNA+54] − for the equimolar mixture. The m / z of 54 corresponds to the mass difference between Fe 2+ and two protons. No multimeric DNA complexes were observed. This result shows that the conjugate, terpy 2 –DNA, does not form intermolecular multimeric complexes, but intramolecularly forms the complex [Fe(terpy) 2 ] 2+ . Metallo-regulation of thermal stability of the duplexes The melting behaviour was studied for the duplexes consisting of the terpy 2 –DNA conjugates and the complementary DNA, ctmp . The ultraviolet melting curves of the duplexes, tp 2 tmp1/ctmp and tp 2 tmp2/ctmp , recorded in the presence of the divalent transition metal ions are shown in Fig. 4 . The melting curves of tp 2 tmp1/ctmp were scarcely affected by any transition metal ions ( Fig. 4a ). In contrast, the duplex structure of tp 2 tmp2/ctmp was apparently stabilized by the addition of an equimolar amount of transition metal ions ( Fig. 4b ). In addition, the metal ions appeared to change the shape of the melting curves of tp 2 tmp2/ctmp to be more cooperative, indicating that the two sequences outside of the terpys cooperatively dissociated in a narrow temperature range in the presence of the metal ions. 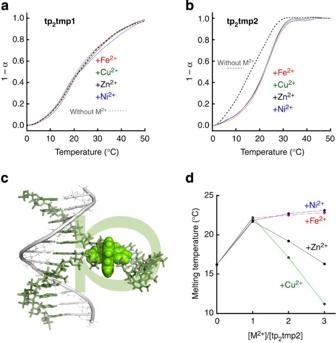Figure 4: Effects of the transition metal ions on melting behaviour of the duplex, terpy2–DNA/ctmp. (a) Ultraviolet melting curves oftp2tmp1/ctmpin the presence of divalent transition metal ions. The dotted curve was obtained in the absence of any transition metals. Red, green, black and blue curves show the melting curves obtained in the presence of Fe2+, Cu2+, Zn2+and Ni2+, respectively. (b) Ultraviolet melting curves oftp2tmp2/ctmpin the presence of divalent transition metal ions. Assignment of the curves are the same witha. Melting experiments were carried out for 1.0 μM DNAs and the metal ions in HEPES buffer solution (10 mM, pH 7.0). (c) One of the possible structures of the Ω-shape DNA duplex,tp2tmp2·Fe2+/ctmp. The model was geometry-optimized by AMBER* force field with GB/SA (generalized Born/surface area) solvent model using MacroModel version 9.5. (d) The effect of the feeding ratio of the metal ions on the melting temperatures of the duplex,tp2tmp2/ctmp. Figure 4: Effects of the transition metal ions on melting behaviour of the duplex, terpy 2 –DNA/ctmp. ( a ) Ultraviolet melting curves of tp 2 tmp1 / ctmp in the presence of divalent transition metal ions. The dotted curve was obtained in the absence of any transition metals. Red, green, black and blue curves show the melting curves obtained in the presence of Fe 2+ , Cu 2+ , Zn 2+ and Ni 2+ , respectively. ( b ) Ultraviolet melting curves of tp 2 tmp2 / ctmp in the presence of divalent transition metal ions. Assignment of the curves are the same with a . Melting experiments were carried out for 1.0 μM DNAs and the metal ions in HEPES buffer solution (10 mM, pH 7.0). ( c ) One of the possible structures of the Ω-shape DNA duplex, tp 2 tmp2 ·Fe 2+ / ctmp . The model was geometry-optimized by AMBER* force field with GB/SA (generalized Born/surface area) solvent model using MacroModel version 9.5. ( d ) The effect of the feeding ratio of the metal ions on the melting temperatures of the duplex, tp 2 tmp2 / ctmp . Full size image The highly cooperative melting behaviour also suggests that [Fe(terpy) 2 ] 2+ observed in ultraviolet–vis titration for tp 2 tmp2 was an intramolecular complex formed on tp 2 tmp2 ·Fe 2+ . That is, tp 2 tmp2 formed an Ω-shaped conformation through intramolecular 1:2 complexation and, concomitantly, the distal two segments located outside of two terpys came close in proximity with each other to form a continuous stretch of the complementary sequence for ctmp ( Fig. 4c ). The duplexes would be stabilized by entropic benefit through metal ion-directed global conformational change of DNA. This could be regarded as dynamic sequence edition. Meanwhile, the complex formation does not affect the global conformation of tp 2 tmp1 , because each of the terpys binds Fe 2+ independently, which is the reason the metal ions scarcely stabilize the duplex tp 2 tmp1/ctmp . The melting temperature of czym/ctmp was 38 °C under the same conditions. Although the Ω-shaped conformation of tp 2 tmp2 ·Fe 2+ gave the same sequence with czym , the duplex stability of tp 2 tmp2 ·Fe 2+ /ctmp did not come up to czym/ctmp . The structure of tp 2 tmp2 ·Fe 2+ could be improved for its structural continuity. Comparable results were commonly observed for chemical ligation products with non-natural structures at the connecting points [37] . It could be improved by optimization of the linker chain structure of terpy units in terpy 2 –DNA. At the point of equimolar ratio ([M 2+ ]/[ tp 2 tmp2 ]=1), all transition metal ions used in the melting study stabilized the duplex tp 2 tmp2/ctmp to a similar extent. However, the dependences of the stabilization effects on the feeding ratio were different for each of the metal ions. For Fe 2+ and Ni 2+ , the duplex remained stable at [M 2+ ]/[ tp 2 tmp2 ]=2 and 3. In contrast, the duplex was destabilized at higher feeding ratios for Cu 2+ and Zn 2+ ( Fig. 4d ). The results essentially coincide with those obtained in the ultraviolet–vis titration. The duplex stability of tp 2 tmp2/ctmp was maintained even in the presence of the excess amount of Fe 2+ and Ni 2+ , because the Ω-shaped conformation of tp 2 tmp2 would be preserved due to the binding properties of the metal ions with terpy, K 1 < K 2 . Meanwhile, for Cu 2+ and Zn 2+ , the global conformation of tp 2 tmp2 would be changed from Ω- to a linear-form accompanying the transition of the complex types formed on tp 2 tmp2 from [M(terpy) 2 ] 2+ (on tp 2 tmp2 ·M 2+ ) to 2[M(terpy)] 2+ (on tp 2 tmp2 ·2M 2+ ) with increasing amounts of the ions due to their magnitudes of the two successive binding constants with terpy, K 1 > K 2 (ref. 36 ). Especially, the binding of Cu 2+ with endocyclic nitrogens of nucleobases is strong [38] , [39] . This would explain the significant inhibition of the duplex formation by Cu 2+ at higher [Cu 2+ ]/[ tp 2 tmp2 ] ratios. Allosteric regulation of DNAzyme activity We constructed the two systems to regulate the activity of DNAzyme by specific coordination of metal ions. The active form of the DNAzyme is a G-quadruplex (G4) structure that requires a hemin as a cofactor [31] , [32] . The catalytic activity was monitored by oxidation of ABTS (2,2′-Azino-bis(3-ethylbenzothiazoline-6-sulphonic acid), which shows green in colour after oxidation [40] . 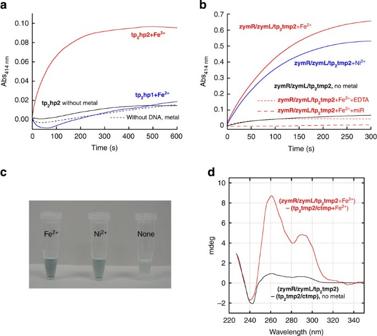Figure 5: Metal ion-directed regulation of DNAzyme activity. (a) Time courses of the ABTS oxidation bytp2hp1andtp2hp2in the presence of Fe2+. The dotted curve was obtained without the conjugates in the absence of any transition metals. Solid curves show the reaction profiles obtained in the presence of the DNA conjugates. Blue:tp2hp1+Fe2+; red:tp2hp2+Fe2+, black:tp2hp2, no metal ions. (b) Time courses of the ABTS oxidation by the split DNAzyme withtp2tmp2in the presence of Fe2+and Ni2+and the effects of reaction inhibitors. Red:zymR/zymL/tp2tmp2+Fe2+; blue:zymR/zymL/tp2tmp2+Ni2+; black:zymR/zymL/tp2tmp2, no metal ions; red dotted:zymR/zymL/tp2tmp2+Fe2++EDTA; red broken:zymR/zymL/tp2tmp2+Fe2++cDNA to the loop region (miR). Typical reaction profiles are shown inaandb. The errors in repetitive reactions were within 10% (s.d.,n=3). DNA complexes (all DNA components:zymR,zymL,tp2hp1,tp2hp2, tp2tmp1andtp2tmp2), 0.40 μM; hemin, 2.0 μM; MCl2, 0.40 μM; H2O2, 2.0 mM; ABTS, 100 μM; HEPES, 14 mM (pH 7.0); NaCl, 700 mM; KCl, 140 mM. (c) Images of reaction solutions shown inb. (d) Differential circular dichroism (CD) spectra of the ternary complex,zymR/zymL/tp2tmp2. Red: (zymR/zymL/tp2tmp2+Fe2+)—(tp2tmp2/ctmp+Fe2+), black: (zymR/zymL/tp2tmp2)—(tp2tmp2/ctmp). CD spectra were measured for 3.0 μM DNAs and the metal ions in HEPES buffer solution (20 mM, pH 7.0) containing 1,000 mM NaCl, 200 mM KCl at 15 °C. Figure 5a shows the time course of the reaction profiles for the conjugates, tp 2 hp1 or tp 2 hp2 , in the presence of an equivalent amount of Fe 2+ . The activity of tp 2 hp2 was apparently restored by Fe 2+ . Such activation was not observed for tp 2 hp1 . As expected from the preliminary studies mentioned above, only tp 2 hp2 seemed to adopt a hairpin structure by intramolecular [Fe(terpy) 2 ] 2+ formation and restored the active form of DNAzyme ( Fig. 1c ). The conjugate tp 2 hp2 could be regarded as a semi-artificial metallo-DNAzyme. However, the activity level of tp 2 hp2 ·Fe 2+ was very little compared with the system of tp 2 tmp2 . The G4-structure formed on tp 2 hp2 ·Fe 2+ might not be ideal as a catalyst. This could be improved by fine-tuning of the structures around terpys. Figure 5: Metal ion-directed regulation of DNAzyme activity. ( a ) Time courses of the ABTS oxidation by tp 2 hp1 and tp 2 hp2 in the presence of Fe 2+ . The dotted curve was obtained without the conjugates in the absence of any transition metals. Solid curves show the reaction profiles obtained in the presence of the DNA conjugates. Blue: tp 2 hp1 +Fe 2+ ; red: tp 2 hp2 +Fe 2+ , black: tp 2 hp2 , no metal ions. ( b ) Time courses of the ABTS oxidation by the split DNAzyme with tp 2 tmp2 in the presence of Fe 2+ and Ni 2+ and the effects of reaction inhibitors. Red: zymR / zymL / tp 2 tmp2 +Fe 2+ ; blue: zymR / zymL / tp 2 tmp2 +Ni 2+ ; black: zymR / zymL / tp 2 tmp2 , no metal ions; red dotted: zymR / zymL / tp 2 tmp2 +Fe 2+ +EDTA; red broken: zymR / zymL / tp 2 tmp2 +Fe 2+ +cDNA to the loop region ( miR ). Typical reaction profiles are shown in a and b . The errors in repetitive reactions were within 10% (s.d., n =3). DNA complexes (all DNA components: zymR , zymL , tp 2 hp1 , tp 2 hp2, tp 2 tmp1 and tp 2 tmp2 ), 0.40 μM; hemin, 2.0 μM; MCl 2 , 0.40 μM; H 2 O 2 , 2.0 mM; ABTS, 100 μM; HEPES, 14 mM (pH 7.0); NaCl, 700 mM; KCl, 140 mM. ( c ) Images of reaction solutions shown in b . ( d ) Differential circular dichroism (CD) spectra of the ternary complex, zymR / zymL / tp 2 tmp2 . Red: ( zymR / zymL / tp 2 tmp2 +Fe 2+ )—( tp 2 tmp2/ctmp +Fe 2+ ), black: ( zymR / zymL / tp 2 tmp2 )—( tp 2 tmp2/ctmp ). CD spectra were measured for 3.0 μM DNAs and the metal ions in HEPES buffer solution (20 mM, pH 7.0) containing 1,000 mM NaCl, 200 mM KCl at 15 °C. Full size image Another allosteric system was also tested to control the activity of DNAzyme. Here tp 2 tmp2 was used as the tunable template to activate the split DNAzyme ( zymR and zymL ) as shown in Fig. 1d . The time course of the reaction profiles is shown in Fig. 5b . Equivalent concentrations of Fe 2+ and Ni 2+ restored the activity of the split DNAzyme in the presence of tp 2 tmp2 . The effect of metal ions could be observed by naked eyes ( Fig. 5c ). The regained activity level was comparable to that of the positive control, zymR / zymL/czym (see Supplementary Fig. 6 ). Cu 2+ and Zn 2+ also showed moderate effect in restoration of split DNAzyme activity (see Supplementary Fig. 5 ). As we expected, global conformation of tp 2 tmp2 was fixed to a Ω-shape by intramolecular formation of [M(terpy) 2 ] 2+ . Then, tp 2 tmp2 ·M 2+ worked as an effective template to reconstruct the integrated active form of DNAzyme. The activity was almost completely suppressed by a large excess amount of EDTA and an equimolar amount of the single-stranded 23-mer DNA ( miR ) with an miR-34 sequence, which is complementary to the loop sequence ( Fig. 5b ). The results of these inhibition experiments confirmed our scheme for the regulation of DNAzyme activity. EDTA removed Fe 2+ from the complex as a masking reagent. The single-stranded DNA with the miR-34 sequence straightened the loop region of tp 2 tmp2 by hybridization and made it impossible to form [Fe(terpy) 2 ] 2+ . The ternary DNA complex zymR / zymL / tp 2 tmp2 was subjected to circular dichroism (CD) spectroscopy. Figure 5d shows the differential CD spectra. To show only the contribution of the DNAzyme moiety, the CD spectrum of tp 2 tmp2/ctmp (duplex+loop) was subtracted from those of zymR / zymL / tp 2 tmp2 (reconstituted DNAzyme+duplex+loop) obtained in the absence and in the presence of Fe 2+ . The characteristic CD band for the mixed-type G4-structure (or the mixture of parallel and antiparallel folded species) was induced by the addition of Fe 2+ (refs 41 , 42 ). This suggests that Fe 2+ activated the DNAzyme by induction of a valid higher-ordered structure through sequence edition of the template, tp 2 tmp2 . Our aim in this study was to induce a drastic conformational change of global DNA (secondary) structure and its application for the allosteric regulation of the function of nucleic acids by certain stimuli. Although several stimuli-responsive DNA conjugates that change their local conformation have been reported [43] , [44] , [45] , the systems of allosteric control of the global DNA structures are quite limited [9] , [17] , [46] , [47] . Even more, as far as we know, there is no precedent of conformational modulation of DNA aiming at sequence edition. The formation of a Ω-shape structure by intramolecular interaction between two specific points on a sequence could be regarded as stimuli-responsive artificial splicing. That is, the distal two segments are directly connected with each other by clipping out the intervening loop sequence. In this study, the specific coordination of terpys to transition metal ions was chosen as a connecting reaction to show the availability of a Ω-motif for regulation of DNA function. Actually, while the phosphates in DNA backbone and nucleobases can coordinate to the transition metal ions [39] , the ions, especially Fe 2+ and Ni 2+ , selectively bind two terpys to form a Ω-shaped structure under experimental conditions. The common preference in coordination chemistry of terpy was retained even for complexation on DNA. Therefore, the Ω-shape structure formation could be designed based on general knowledge in coordination chemistry. The kind and concentration of the metal ions, the structure of the terpy and the design of the conjugate architecture could be effective factors to control the system. Especially, it was interesting that local structural differences (just as ≈1.4 Å) in terpy units, such as substitution positions, were critically important to define the global structure. We succeeded in the regulation of DNAzyme activity using the Ω-motif. Judging from the results of ultraviolet–vis titration, ultraviolet melting, CD spectroscopy, modelling analysis by DFT and ABTS oxidation and inhibition experiments, the activity of DNAzyme was regulated basically according to the proposed scheme shown in Fig. 1 . However, the difference in melting temperatures of the duplex tp 2 tmp2/ctmp observed in the presence and absence of Fe 2+ might not be enough to solely explain the sharp response in restoration of DNAzyme activity. At least, the CD spectra showed that Fe 2+ induced the active G4-structure of DNAzyme. Fe 2+ could work as an essential factor not only to assemble the split DNAzymes but also to induce the active G4-structure through complexation. To construct the system for artificial (non-enzymatic or chemical) splicing of DNA, we can choose appropriate clipping reactions from many bioorthogonal chemistries including click reactions [48] , [49] and photochemical reactions [37] , [44] , [45] , [46] , [50] . The techniques could be applied for signal amplification in bioanalyses through DNA circuits based on autonomous succession of strand exchange [26] , [51] . The regulation of cell function through the control of gene expression would also be very compatible and a promising application. Synthesis Preparation [30] of the amidite reagents, 1 and 2 , and DNAs are described in the Supplementary Information . Ultraviolet–vis titration The aliquots (typically, 0.40 μl) [16] , [52] , [53] of a 0.50mM stock solution of MCl 2 (M=Fe 2+ , Ni 2+ , Cu 2+ or Zn 2+ ) were titrated into a 1.0ml solution of 2.0 μM DNA or DNA complex ( tp 2 tmp1 , tp 2 tmp2 , tp 2 tmp1 / ctmp or tp 2 tmp2 / ctmp , in 10 mM HEPES (pH 7.0), 500 mM NaCl) in a cuvette, and then the solution was mixed well. The ultraviolet–vis spectra were measured using a spectrophotometer V-650 (Jasco) at 25 °C, after 30 min incubation following each addition. Ultraviolet melting Thermal denaturation experiments were performed [9] , [54] , [55] in HEPES buffer solution (10 mM, pH 7.0) on a UV-1650 (Shimadzu) ultraviolet–vis spectrophotometer equipped with a Peltier thermal controller. Concentrations of each DNA strand and MCl 2 (M=Fe 2+ , Ni 2+ , Cu 2+ or Zn 2+ ) were 1.0 μM. Prior to the beginning of each melt, the samples were degassed at 85 °C for 5 min and then annealed by slowly cooling to 0 °C. In the denaturation experiments, the solutions were heated at a rate of 0.5 deg min −1 after equilibration for 20 min at 0 °C. The temperature that gave the maximum first derivative of the melting curve was used as the melting temperature, a measure of the thermal stability of the duplexes. Circular dichroism measurement CD [56] , [57] spectra were measured in HEPES buffer solution (20 mM, pH 7.0) containing 1.0 M NaCl and 200 mM KCl on a J-725 Spectropolarimeter (Jasco) equipped with a Peltier thermal controller, at 15 °C. Concentrations of all DNA strands and FeCl 2 were 3.0 μM. Prior to the beginning of each melt, the samples were degassed at 85 °C for 5 min and then annealed by slowly cooling to 15 °C. To only show the contribution of the DNAzyme moiety, the CD spectrum of tp 2 tmp2/ctmp (duplex+loop) was subtracted from those of zymR / zymL / tp 2 tmp2 (reconstituted DNAzyme+duplex+loop) obtained in the absence and in the presence of Fe 2+ . Molecular modelling Both complex ([Fe(terpy) 2 ] 2+ ) structures were calculated by the DFT method (B3LYP/6-31G*) using Spartan 10 (Wavefunction Inc., USA). The molecular models shown in Fig. 4c were constructed with MacroModel (ver. 9.5, Schrödinger Inc., USA). The initial structure was built as a standard double helix using the Maestro (Schrödinger Inc.) fragment library. The optimization was performed with an AMBER* force field with generalized Born/surface area treatment of solvation. Allosteric catalytic reactions by split DNAzymes Into the mixed solution of DNA and hemin, [40] , [58] , [59] was added the solution containing MCl 2 (M=Fe 2+ , Ni 2+ , Cu 2+ or Zn 2+ ), H 2 O 2 and ABTS to prepare 1.0 ml of the reaction solution in a cuvette. The final concentrations of each of the components were as follows: DNA complexes (all DNA components: zymR , zymL , czym , tp 2 hp1 , tp 2 hp2, tp 2 tmp1 and tp 2 tmp2 ), 0.40 μM; hemin, 2.0 μM; MCl 2 , 0.40 μM; H 2 O 2 , 2.0 mM; ABTS, 100 μM; HEPES, 14 mM (pH 7.0); NaCl, 700 mM; KCl, 140 mM. The progress of ABTS oxidation was monitored at 15 °C by the change in absorbance at 414 nm. The time courses of absorbance change were monitored using a spectrophotometer V-650 (Jasco) equipped with a Peltier thermal controller. How to cite this article: Ihara T. et al. Metal ion-directed dynamic splicing of DNA through global conformational change by intramolecular complexation. Nat. Commun. 6:6640 doi: 10.1038/ncomms7640 (2015).